The saccus vasculosus of fish is a sensor of seasonal changes in day length The pars tuberalis of the pituitary gland is the regulatory hub for seasonal reproduction in birds and mammals. Although fish also exhibit robust seasonal responses, they do not possess an anatomically distinct pars tuberalis. Here we report that the saccus vasculosus of fish is a seasonal sensor. We observe expression of key genes regulating seasonal reproduction and rhodopsin family genes in the saccus vasculosus of masu salmon. Immunohistochemical studies demonstrate that all of these genes are expressed in the coronet cells of the saccus vasculosus, suggesting the existence of a photoperiodic signalling pathway from light input to neuroendocrine output. In addition, isolated saccus vasculosus has the capacity to respond to photoperiodic signals, and its removal abolishes photoperiodic response of the gonad. Although the physiological role of the saccus vasculosus has been a mystery for several centuries, our findings indicate that the saccus vasculosus acts as a sensor of seasonal changes in day length in fish. Animals living outside the tropics use changes in the photoperiod to adapt to seasonal changes in the environment, a phenomenon so-called photoperiodism. Recent studies have uncovered the signal transduction pathway regulating photoperiodism in birds and mammals. The pars tuberalis (PT) of the pituitary gland and the ependymal cells lining ventrolateral walls of the third ventricle within the mediobasal hypothalamus are considered to have critical roles in the regulation of photoperiodism in both birds and mammals [1] , [2] , [3] . Long-day (LD)-induced thyrotropin (thyroid-stimulating hormone (TSH)) within the PT, a master factor regulating seasonal reproduction, acts on the TSH receptor (TSHR) on the ependymal cells to induce DIO2 expression. DIO2 encodes type 2 iodothyronine deiodinase, a thyroid hormone-activating enzyme, which converts prohormone thyroxine (T 4 ) to bioactive 3,3′,5-triiodothyronine (T 3 ). LD-induced T 3 induces morphological changes between gonadotropin-releasing hormone nerve terminals and endfeet of glial processes, and these changes in the neuro–glial interaction appear to regulate seasonal gonadotropin-releasing hormone secretion from the median eminence to the portal capillary, and hence gonadotropin secretion from the pituitary gland [4] , [5] . Although the downstream mechanism of PT-derived TSH appears to be conserved, the light-input pathway regulating TSH in the PT is completely different between birds and mammals. In mammals, eyes are the only photoreceptive organs, and photoperiodic information received by the eye is transmitted to the pineal organ through the suprachiasmatic nucleus, which serves as the circadian pacemaker. Length of night is encoded by the duration of melatonin secretion from the pineal organ [6] , and melatonin suppresses expression of TSH through the MT1 melatonin receptor in the PT [2] , [7] . In birds, by contrast, melatonin has little effect on photoperiodic response of gonads [8] . Furthermore, neither eyes nor the pineal organ, another photoreceptive organ in non-mammalian vertebrates, are necessary for the photoperiodic response in birds [9] ; instead, light received by the deep-brain photoreceptors induces expression of TSH in the PT [10] . Most fish living outside the tropics also exhibit a photoperiodic response [11] , and involvement of thyroid hormone in the regulation of seasonal reproduction has been described extensively [12] . However, fish do not possess an anatomically distinct PT, which is the regulatory hub of photoperiodism in birds and mammals. Here, we seek to identify the photoperiodic centre in fish using short-day (SD)-breeding masu salmon ( Oncorhynchus masou masou ) [13] , and find that the saccus vasculosus (SV) is the sensor of seasonal changes in day length in fish. Expression of key genes regulating photoperiodism in the SV Underyearling precocious male masu salmon kept under natural light conditions in Nikko, Tochigi, Japan (36.44°N), were divided into two groups. One group was transferred into an SD condition (8 h light, 16 h dark: 8L16D; 4:00 light on, 12:00 light off), and the other group was transferred into an LD condition (16L8D; 4:00 light on, 20:00 light off). Temperature was kept at 9–10 °C during the experiment, and the daily feeding rations were set at 2% of body weight. Brains were collected 8 weeks after the fish were transferred into each light condition. When we examined the expression of key genes involved in the regulation of the photoperiodic response, we observed a robust photoperiodic response of DIO2 in the SV ( Fig. 1a–e ). The SV is a specialised circumventricular organ found in the caudal hypothalamus of many jawed fish, but its physiological function remains unclear [14] , [15] , [16] . Biological activity of TSH requires heterodimerization of the TSH β-subunit and a common glycoprotein α-subunit. Although the TSHB (encoding the β-subunit of TSH), CGA (common glycoprotein α-subunit) and TSHR genes were expressed in the SV, and their expression exhibited tendencies similar to that of DIO2 , we did not observe statistically significant differences in the expression of these genes between the SD and LD conditions ( Fig. 1d ). No hybridization signal was observed in the control ( Supplementary Fig. S1 ). 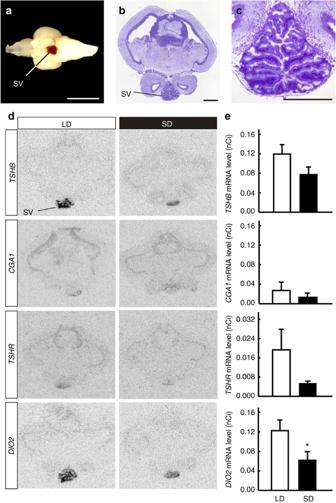Figure 1: Expression of key genes regulating seasonal reproduction in the SV. (a) Ventral view of the masu salmon (O. masou masou) brain. Rostral is to the left. (b,c) Nissl-stained coronal section of the brain (b) and enlarged picture of the SV (c). (d,e) Effect of changing day length on expression ofTSHB,CGA1,TSHRandDIO2in the SV examined byin situhybridization. Fish were exposed to 8 weeks of LD or SD conditions. *P<0.05 (t-test) (mean+s.e.m.,n=5). Scale bars, 5 mm (a); 1 mm (b); and 500 μm (c). Figure 1: Expression of key genes regulating seasonal reproduction in the SV. ( a ) Ventral view of the masu salmon ( O. masou masou ) brain. Rostral is to the left. ( b , c ) Nissl-stained coronal section of the brain ( b ) and enlarged picture of the SV ( c ). ( d,e ) Effect of changing day length on expression of TSHB , CGA1 , TSHR and DIO2 in the SV examined by in situ hybridization. Fish were exposed to 8 weeks of LD or SD conditions. * P <0.05 ( t -test) (mean+s.e.m., n =5). Scale bars, 5 mm ( a ); 1 mm ( b ); and 500 μm ( c ). Full size image Expression of rhodopsin family genes in the SV More than a hundred years ago, Karl von Frisch [17] demonstrated evidence for the existence of deep-brain photoreceptors in fish. However, the localization and identity of these deep-brain photoreceptors are not entirely known. Therefore, we performed a comprehensive expression analysis of gene encoding rhodopsin family members in the brain, as well as in the eye and pineal organ. Within the retina, we observed strong expression of rhodopsin ( RH1 ), short wavelength-sensitive opsin 1 ( SWS1 ), short wavelength-sensitive opsin 2 ( SWS2 ), middle wavelength-sensitive opsin 2A ( RH2A ) and long wavelength-sensitive opsin ( LWS ), as well as weak expression of middle wavelength-sensitive opsin 2B ( RH2B ) and melanopsin ( OPN4 ) ( Supplementary Fig. S2 ). We also observed strong expression of exorhodopsin ( EXORH ) and SWS1 , and weak expression of SWS2 and parapinopsin B ( PP ) in the pineal organ ( Supplementary Fig. S3 ). In the SV, we observed expression of four opsin genes ( RH1 , SWS1 , LWS and OPN4) ( Fig. 2 , Supplementary Fig. S4 ). 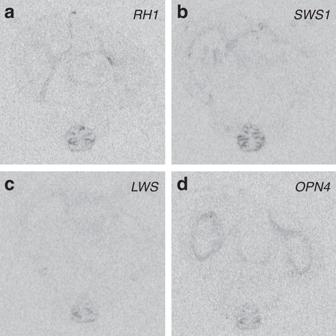Figure 2: Expression of rhodopsin family genes in the SV. Representative autoradiograms for expression of opsin genes. (a)RH1: rhodopsin; (b)SWS1: short wavelength-sensitive opsin 1; (c)LWS: long wavelength-sensitive opsin; and (d)OPN4: melanopsin. Figure 2: Expression of rhodopsin family genes in the SV. Representative autoradiograms for expression of opsin genes. ( a ) RH1 : rhodopsin; ( b ) SWS1 : short wavelength-sensitive opsin 1; ( c ) LWS : long wavelength-sensitive opsin; and ( d ) OPN4 : melanopsin. Full size image Coronet cells contain photoperiodic signalling pathway To further examine the detailed localization of the aforementioned genes, we attempted to raise antibodies against TSHβ, DIO2, RH1, SWS1, LWS and OPN4. Among these, we succeeded in generating specific antibodies against TSHβ, DIO2, SWS1 and OPN4 ( Fig. 3 , Supplementary Fig. S5 ). We performed western blot analysis on tissues previously demonstrated to express each of these genes, and observed single specific bands at the expected molecular sizes ( Supplementary Fig. S5 ). TSHβ was observed in the adenohypophysis ( Supplementary Fig. S5a,b ), DIO2 in the gill ( Supplementary Fig. S5c,d ), SWS1 in the outer segments of photoreceptors ( Supplementary Fig. S5f ) and OPN4 in the ganglion cells of the retina ( Supplementary Fig. S5h ). All of these signals were eliminated by preadsorption of the antibodies with an excess amount of the corresponding antigenic peptide ( Supplementary Fig. S5 ). The SV consists of three types of cells: coronet (crown) cells, cerebrospinal fluid (CSF)-contacting cells and supporting cells. Coronet cells are characterized by an apical crown of globule-tipped cilia protruding into the ventricle [16] ( Fig. 3a ), whereas the CSF-contacting neurons are bipolar neurons with a knob-like structure; their morphology resembles that of photoreceptor cells in the developing retina [18] . In a previous study, we demonstrated that OPN5-positive CSF-contacting neurons in the quail hypothalamus are a type of deep-brain photoreceptors that mediate the photoperiodic response [10] . Therefore, we predicted that opsins would be expressed in CSF-contacting neurons in the SV. Unexpectedly, however, SWS1 and OPN4 were expressed in the globules of the coronet cells ( Fig. 3b ). Interestingly, TSHβ were also observed in the globules of coronet cells, whereas DIO2 were observed in the protrusions and apical regions of the cell bodies of coronet cells ( Fig. 3b ). These results were further confirmed by immunoelectron microscopy ( Fig. 3c ). We confirmed expression of DIO2 in the protrusion, and SWS1 and OPN4 in the globules, consistent with the results of light-microscopic immunohistochemistry. (We failed to detect TSHβ owing to the lower sensitivity of immunoelectron microscopy relative to immunohistochemistry.) These results suggest that coronet cells in the SV contain entire photoperiodic signalling pathway from light input (photoreceptor) to neuroendocrine output (TSHβ and DIO2). The coronet cells have traditionally been considered to be responsible for the function of the SV [14] , [15] , [16] , and our results are consistent with this notion. As the circadian clock is involved in photoperiodic time measurement, we also examined and confirmed expression of circadian clock genes in the SV ( Supplementary Fig. S6 ). The detailed localization and temporal expression profiles of clock proteins remain to be clarified in future studies. 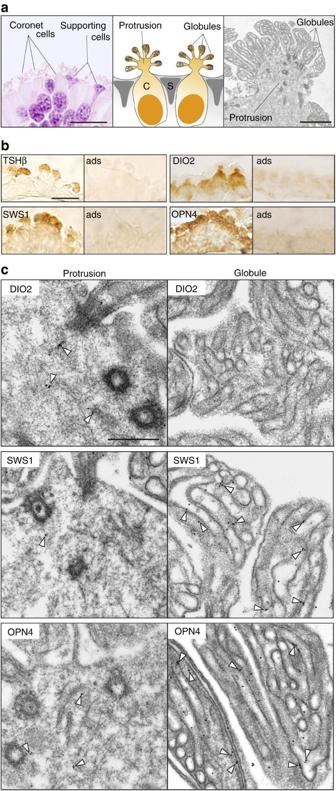Figure 3: Localization of regulatory components of photoperiodism in the coronet cells. (a) Morphology of coronet cells. Left: hematoxylin–eosin (H–E) stain. Centre: schematic drawing. C, coronet cell; S, supporting cell. Right: electron microscopic image. (b,c) Representative photomicrograph of immunohistochemistry (b) and immunoelectron microscopic analysis (c) for TSHβ, DIO2, SWS1 and OPN4. Signals were eliminated when antibodies were pre-adsorbed (ads) with an excess of the corresponding antigenic peptides. Scale bars, (a) left: 10 μm; right: 2 μm; (b) 10 μm; (c) 500 nm. Figure 3: Localization of regulatory components of photoperiodism in the coronet cells. ( a ) Morphology of coronet cells. Left: hematoxylin–eosin (H–E) stain. Centre: schematic drawing. C, coronet cell; S, supporting cell. Right: electron microscopic image. ( b , c ) Representative photomicrograph of immunohistochemistry ( b ) and immunoelectron microscopic analysis ( c ) for TSHβ, DIO2, SWS1 and OPN4. Signals were eliminated when antibodies were pre-adsorbed (ads) with an excess of the corresponding antigenic peptides. Scale bars, ( a ) left: 10 μm; right: 2 μm; ( b ) 10 μm; ( c ) 500 nm. Full size image Isolated SV responds to photoperiodic changes To further examine whether the SV itself has the capacity to respond to photoperiodic changes, we exposed organ-cultured SV to SD or LD conditions for 1 week. We observed a photoperiodic response in TSHβ and DIO2 protein levels ( Fig. 4a–c , Supplementary Fig. S7 ), indicating that the isolated SV is a photoperiodic sensor. Both TSHβ and DIO2 appeared to exhibit circadian variation, as has also been reported in hamster [19] . However, despite the changes in protein levels, we did not observe significant changes in the corresponding messenger RNA levels by real-time quantitative PCR (Q-PCR) ( Fig. 4d ). When we examined protein and mRNA levels in the SV of fish exposed to SD and LD conditions for 5 weeks, protein levels showed marked changes, whereas mRNA levels did not differ ( Supplementary Fig. S8 ). Daily rhythm of melatonin is regulated by the rate-limiting enzyme arylalkylamine N -acetyltransferase (AA-NAT) in the pineal organ. Although AA-NAT mRNA levels exhibit daily rhythms in most species examined, rainbow trout ( Oncorhynchus mykiss ) is the exception. In the trout, AA-NAT2 mRNA levels exhibit little change, and the melatonin rhythm is considered to be dependent on a posttranscriptional mechanism [20] . Such a posttranscriptional mechanism may be more important than transcriptional regulation in several physiological events in the genus Oncorhynchus . As we observed a photoperiodic difference in DIO2 mRNA at 8 weeks after the transfer from LD to SD conditions ( Fig. 1 ), transcriptional regulation appears to happen later. 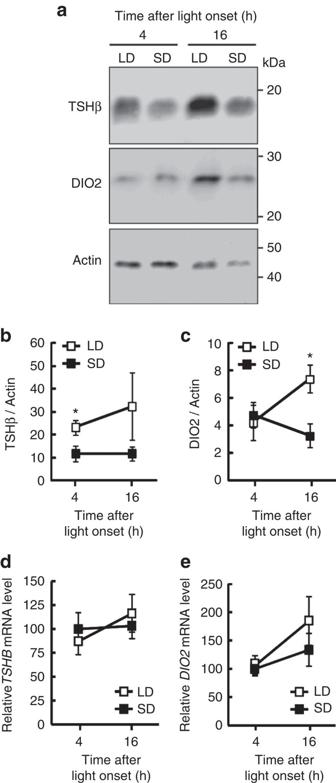Figure 4: Isolated SV has the capacity to respond to photoperiodic signals. (a–c) Isolated SV was cultured under SD and LD conditions, and western blot analysis (a–c) and Q-PCR (d,e) were performed. Although photoperiodic responses of TSHβ and DIO2 were observed at the protein level (a–c), no significant differences were observed in their mRNA levels (d,e) (t-test, *P<0.05, mean±s.e.m.,n=4–6). Figure 4: Isolated SV has the capacity to respond to photoperiodic signals. ( a–c ) Isolated SV was cultured under SD and LD conditions, and western blot analysis ( a–c ) and Q-PCR ( d,e ) were performed. Although photoperiodic responses of TSHβ and DIO2 were observed at the protein level ( a–c ), no significant differences were observed in their mRNA levels ( d,e ) ( t -test, * P <0.05, mean±s.e.m., n =4–6). Full size image Removal of the SV abolishes photoperiodic response Thyroid hormone is involved in the regulation of seasonal reproduction in fish. Positive correlations between various thyroidal indices and reproductive status have been reported in the majority of seasonally breeding teleosts, and thyroidal activity increases during early gonadal development [12] . In addition, radiothyroidectomy results in a major inhibition of testicular development, which can be rescued by thyroid hormone treatment [21] . Furthermore, inhibition of thyroid hormone secretion by thiourea also inhibits early testicular development [22] . To further examine the involvement of the SV in the photoperiodic response in vivo , we have examined the effect of SV removal (SVX) on the photoperiodic response of the gonad in underyearling male masu salmon. We removed the SV using the transorbital surgical technique described by Nishioka et al . [23] . SVX was performed in a total of 150 fish. Among them, 68 fish survived, and these fish were divided into two groups and exposed to 5 weeks of SD (8L16D; 4:00 light on, 12:00 light off) or LD (16L8D; 4:00 light on, 20:00 light off) conditions at 18–19 °C in Hitachiota, Ibaraki, Japan (36.43°N), respectively. Post-mortem examination revealed that the SV removal was successful in six fish (four fish in the SD group and two fish in the LD group). In these fish, other brain regions (for example, hypothalamus and pituitary) were intact. Fish with SV fragments (partial SVX) or SVX fish with damaged brains were eliminated from the analysis. Body weight was significantly smaller in sham-operated and SVX fish than in intact fish under SD conditions ( Fig. 5a ; Kruskal–Wallis test, P <0.01, Steel–Dwass post-hoc test, P <0.05; n =4–10), and a similar tendency was also observed under LD conditions ( Supplementary Fig. S9a ). Smaller body weight in sham-operated and SVX fish appeared to be the result of unilateral orbital enucleation. However, we cannot exclude the possibility that the SV is involved in the growth of masu salmon. Under LD conditions, the gonadosomatic index (weight of gonad relative to body weight: GSI) and plasma testosterone were low in all groups of fish ( Supplementary Fig. S9b,c ). By contrast, significant increases in GSI and plasma testosterone were observed in intact and sham-operated fish under SD conditions ( Fig. 5b ). However, such an increase was not observed in SVX fish. These results suggest that the SV is involved in the photoperiodic regulation of the gonad in the masu salmon. LD stimulus is known to induce TSH release from the PT in both LD- and SD-breeding birds and mammals, suggesting that PT-derived TSH is the ‘springtime hormone’ [1] , [2] , [3] . In this study, we also observed high expression of TSH in the SV of masu salmon under LD conditions. The mechanism that determines the differences between SD and LD breeders appears to act downstream of TSH action, but the underlying mechanisms remain unsettled. 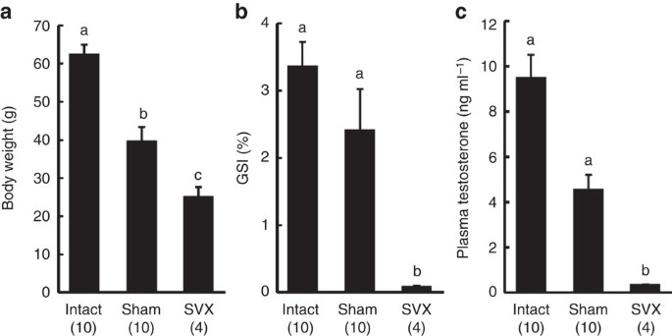Figure 5: Removal of the SV blocks SD-induced testicular growth. Effect of SD stimulus on body weight (a), GSI (b), plasma testosterone (c) was examined in intact, sham-operated and SV-removed (SVX) masu salmon. Numbers in parentheses represent the number of animals used in each group. Different characters indicate significant differences (Kruskal–Wallis test,P<0.01; Steel–Dwasspost-hoctest,P<0.05, mean+s.e.m.,n=4–10). Figure 5: Removal of the SV blocks SD-induced testicular growth. Effect of SD stimulus on body weight ( a ), GSI ( b ), plasma testosterone ( c ) was examined in intact, sham-operated and SV-removed (SVX) masu salmon. Numbers in parentheses represent the number of animals used in each group. Different characters indicate significant differences (Kruskal–Wallis test, P <0.01; Steel–Dwass post-hoc test, P <0.05, mean+s.e.m., n =4–10). Full size image Comparative neurology emerged in the 17th century in England, and the SV was first depicted by Samuel Collins [24] , an anatomist and president of the Royal College of Physicians in 1685 (refs15,25) [15] , [25] . Since then, its existence was confirmed in various species, and Gottsche (1835) [26] named this tissue the ‘saccus vasculosus’ and demonstrated that the SV has secretory function. Thereafter, the SV has been suggested to be involved in sensory and transport functions as well as secretory functions (for example, liquor pressure perception, osmoregulation, calcium homeostasis, glucose loading and transcellular ion exchange between blood vessels and CSF) [15] , [16] , [27] . However, its function has remained mysterious. In this study, we have finally demonstrated that the SV is the organ that regulates photoperiodism in fish. We demonstrated expression of SWS1 and OPN4 in the globules of coronet cells. Although we have tried to generate antibodies against all the opsins expressed in the SV, the specificities of the antibodies we raised against RH1 and LWS were not satisfactory. As the CSF-contacting neuron is the deep-brain photoreceptor in quail [10] , it is reasonable to speculate that some of these opsins may be expressed in CSF-contacting neurons, to act as another type of photoreceptor in the SV. This possibility remains to be examined in a future study. Coronet cells express vimentin and/or glial fibrillary acidic protein, markers of glial cells [28] . We observed expression of DIO2 in coronet cells, which seems reasonable because DIO2 is expressed in the vimentin-positive ependymal cells (also known as tanycytes) lining the ventrolateral walls of the third ventricle in birds and mammals [4] , [29] . In addition to photoreceptive and glial characteristics, coronet cells have been suggested to have endocrine function [15] , [27] . Consistent with this, we demonstrated the localization of TSH in the coronet cells. All of these results suggest that coronet cells have multiple functions, ranging from photoreception to neuroendocrine output, reminding us of the structural and functional evolution of the pineal organ [30] , [31] . In non-mammalian vertebrates, pinealocytes of the pineal organ contain photoreceptors (for detecting light input) and circadian pacemaker (for clock functions), and produce melatonin (neuroendocrine output). However, during the course of evolution, the mammalian pinealocyte has lost the photoreceptive and pacemaker functions and acts primarily as an endocrine organ that secretes melatonin. It has been proposed that multifunctionality (for example, sensory and neurosecretory functions) is a general feature of ancient cell types (Vigh’s protoneuron concept) [32] , [33] , [34] . Over the course of evolution, these multiple functions were then inherited in a complementary manner by sister cell types with increasing specialization. This principle is called ‘segregation of functions’, and may explain the emergence of axonal circuits during the evolution of the nervous system [34] . As the fish coronet cell contains the whole photoperiodic machinery, from the detection of light input to neuroendocrine output, in a single cell, it appears to represent an ancestral photoperiodic sensor. CSF-contacting neurons of the SV are immunoreactive for gamma-aminobutyric acid, glutamic acid decarboxylase and neuropeptide Y [35] (ref.35). However, the functions of CSF-contacting neurons, as well as supporting cells within the SV, remain unknown. In addition, we still do not know why the SV is highly vascularized. Thus, we cannot exclude the possibility that the SV has other physiological functions in addition to serving as the seasonal sensor. Afferent and efferent fibre systems relating the SV and the hypothalamus to each other have been reported [14] , [16] , [27] , [35] . A close developmental relationship between the neurohypophysis and caudal wall of the infundibulum has also been reported [36] . However, very few investigations have been conducted regarding the development of the SV [16] . Therefore, it would be interesting to study the development of SV in the future. Animals Masu salmon ( O. masou masou ) was used in this study, which was approved by the Animal Experiment Committee of Nagoya University and Utsunomiya University. In situ hybridization Non-perfused frozen sections were examined with 33 P-labelled oligonucleotide probes [37] . Hybridization was carried out overnight at 42 °C, and two high-stringency posthybridization washes were performed at 55 °C. The sections were air dried and exposed to BioMax MR film (Eastman Kodak). The probe sequences are shown in Supplementary Table S1 . Antibodies We generated rabbit polyclonal antibodies against masu salmon TSHβ (CSKPLRHIYPYPGLNSYIHPN), DIO2 (CKLGFEAPNSKVVKVPGS), SWS1 (MGKDFHLYENISKVSPFC) and OPN4 (KINEGTRDSVKSMHKMRC). Purified peptides conjugated to keyhole limpet haemocyanin were dissolved in 8 M urea containing 1,3-diaza-2,4-cyclopentadiene (imidazole) and used as an immunogen. After injecting the immunogen into each rabbit six times, blood was collected and IgG molecules were purified using peptide-Sepharose affinity chromatography. Purified antibodies were dialyzed in PBS and concentrated. IgG was stored at −30 °C in PBS containing 50% glycerol. Western blotting Membranes were incubated with primary antibodies overnight at 4 °C. To ascertain the specificity of the immunostaining, immunoadsorption analysis was performed. Antibodies were diluted for western blotting: rabbit anti-TSHβ serum, 1:5,000; anti-DIO2 antibody, 1:200; anti-SWS1 antibody, 1:200; and anti-OPN4 antibody, 1:200; and goat anti-β-actin antibody (Santa Cruz Biotechnology Inc., sc-1616), 1:2,000. Following incubation with anti-rabbit or goat IgG secondary antiserum, immunoreactive bands were visualized by enhanced chemiluminescent detection (ImmunoStar LD, WAKO, Japan), and observed using an LAS-3000 mini imager (Fujifilm, Tokyo, Japan) [38] . Immunohistochemical and immunoelectron microscopic studies Immunohistochemistry was performed using rabbit anti-TSHβ serum (1:5,000), anti-DIO2 (1:200), anti-SWS1 (1:200) and anti-OPN4 (1:200) antibodies, and a Vectastain Elite ABC rabbit IgG kit (Vector Laboratories) with a standard protocol [38] . Immunoelectron microscopic study was performed using post-embedding immunogold labelling technique with gold-tagged (15 nm) goat anti-rabbit IgG polyclonal antibody (1:100) (British Biocell International Ltd.). SV culture The SV was dissected out from masu salmon reared under SD (8L16D; 4:00 light on, 12:00 light off). Dissected SVs were maintained individually in 1 ml of L-15 (Sigma) containing 1X Antibiotic-Antimycotic (Life Technologies) in 24-well plates under either SD or LD (16L8D; 4:00 light on, 20:00 light off) at 15 °C for 7 days. Then, SV were collected at 4 or 16 h after light onset and either immediately immersed in RNAlater (Life Technologies) for Q-PCR or frozen in liquid nitrogen for western blotting. Quantitative PCR Reverse transcription was performed on total RNA (100 ng) using High Capacity cDNA Reverse Transcription Kit (Life Technologies) and random primers. Samples contained 1X LightCycler 480 SYBR Green I Master (Roche), 0.5 μM gene-specific primers ( Supplementary Table S2 ), and 1/5 (for TSHB and DIO2 ) or 1/50 (for ACTB : β-actin) synthesized cDNA in a 5 μl volume. Q-PCR was performed in duplicates using a LightCycler 480 Real-Time PCR System (Roche) as follows: 95 °C for 5 min; 50 cycles of 95 °C for 10 s, 60 °C for 10 s and 72 °C for 10 s; followed by melting curve analysis. We used ACTB as an internal control. Values were expressed as percentage of the value at 4 h after light onset under the SD condition. SV removal Underyearling precocious male masu salmon were anesthetized with 0.1 g l −1 ethyl m -aminobenzoate methanesulfonate (MS-222, Sigma). The SV was removed using the transorbital surgical technique. After removing the right eyes, adipose tissue and blood were removed using cotton swabs. A hole was drilled behind the optic foramen and the SV was aspirated with a 200 μl pipettor inserted through the hole. Unilateral orbital enucleation was performed in the sham-operated fish. Sham-operated control fish were treated identically except for pipettor insertion and aspiration. Testosterone measurement Plasma samples were extracted with diethylether and testosterone levels in the extracts were determined by radioimmunoassay using [ 3 H]-testosterone (PerkinElmer) and anti-testosterone (FKA-206, Cosmo Bio Co. Ltd.) [39] . Parallelism of inhibition curves was proved between serial twofold dilution of testosterone standard and the plasma extract. Statistical analysis Data are presented as means+s.e.m. Normally distributed data were analysed by parametric tests (for example, t -test), and non-normally distributed data were analysed by non-parametric tests (for example, Mann–Whitney U -test and Kruskal–Wallis one-way analysis of variance). How to cite this article: Nakane, Y. et al . The saccus vasculosus of fish is a sensor of seasonal changes in day length. Nat. Commun. 4:2108 doi: 10.1038/ncomms3108 (2013).